The adhesion GPCR Gpr56 regulates oligodendrocyte development via interactions with Gα12/13and RhoA In the vertebrate central nervous system, myelinating oligodendrocytes are postmitotic and derive from proliferative oligodendrocyte precursor cells (OPCs). The molecular mechanisms that govern oligodendrocyte development are incompletely understood, but recent studies implicate the adhesion class of G protein-coupled receptors (aGPCRs) as important regulators of myelination. Here, we use zebrafish and mouse models to dissect the function of the aGPCR Gpr56 in oligodendrocyte development. We show that gpr56 is expressed during early stages of oligodendrocyte development. In addition, we observe a significant reduction of mature oligodendrocyte number and myelinated axons in gpr56 zebrafish mutants. This reduction results from decreased OPC proliferation, rather than increased cell death or altered neural precursor differentiation potential. Finally, we show that these functions are mediated by Gα 12/13 proteins and Rho activation. Together, our data establish Gpr56 as a regulator of oligodendrocyte development. Myelin is a multilamellar, lipid-rich membrane that insulates axons in the vertebrate nervous system to facilitate the rapid conduction of action potentials [1] . In addition, myelinating glia promote neuronal health by providing vital trophic support to the axons they ensheath [2] , [3] . Myelin is generated by specialized glial cells—Schwann cells (SCs) in the peripheral nervous system (PNS) and oligodendrocytes in the central nervous system (CNS) [1] . Oligodendrocytes form the myelin sheath by extending and iteratively wrapping their plasma membranes around axons, while glial cell cytoplasm is extruded to ultimately form compact myelin [4] . Impaired myelination causes debilitating symptoms in many severe neurological disorders such as multiple sclerosis, and loss of mature oligodendrocytes and myelin can lead to neuronal death and eventual paralysis. Therefore, continued research to uncover new pathways that promote oligodendrocyte development and remyelination is essential [5] . Although myelin is required for human life, the molecular mechanisms that underlie glial cell development and myelination are incompletely understood. Previous studies indicate that extracellular matrix proteins and their receptors, in addition to intracellular signal-transduction cascades, are essential for proper development of myelinating glial cells [6] , [7] . For this reason, adhesion G protein-coupled receptors (aGPCRs) represent good candidate regulators of glial cell development and myelination because they are purported to regulate both cell–cell and cell–matrix interactions as well as signal-transduction by heterotrimeric G proteins [8] , and recent studies implicate aGPCRs as important regulators of myelination [9] , [10] , [11] , [12] , [13] . Indeed, the aGPCR Gpr126 is essential for SC, but not oligodendrocyte, myelination [10] , [11] , [12] , [13] . aGPCRs are the second largest class of GPCRs, but remain relatively understudied due to their structural complexity. In addition to the canonical seven-transmembrane (7TM) domain common to all GPCRs that usually facilitates intracellular signalling, aGPCRs are characterized by the presence of a very large N-terminal domain rich in functional motifs associated with cell–cell and cell–matrix adhesion, which is separated from the 7TM by a GPCR proteolytic site (GPS) [14] . The GPS motif is encompassed by a larger GPCR autoproteolysis-inducing (GAIN) domain [15] . Together, these domains are required for autoproteolytic cleavage of the N terminus from the C terminus, a process that may be required for proper intracellular aGPCR trafficking and signalling [15] , [16] . The dual roles of aGPCRs in promoting cell–cell/cell–matrix interactions and facilitating intracellular signalling, in addition to the importance of Gpr126 for SC myelination [10] , [11] , [12] , [13] , led us to hypothesize that additional aGPCRs regulate glial cell development and myelination in the CNS. Previously published data sets indicate that Gpr56 , an aGPCR related to Gpr126, is highly expressed during mouse CNS development in oligodendrocyte precursor cells (OPCs) [17] , [18] . In addition, mutations in GPR56 in humans cause bilateral frontoparietal polymicrogyria (BFPP) [19] , a cortical brain malformation associated with a variety of devastating neurological impairments such as epilepsy and mental retardation. Interestingly, brains of BFPP patients also exhibit reduced white matter volume by MRI [20] , [21] , [22] , indicative of myelin defects. Taken together, these data suggest that Gpr56 may function in oligodendrocyte development. To test this hypothesis, we utilize zebrafish and mouse model systems to explore the necessity of Gpr56 in the CNS. We show that impaired Gpr56 function results in reduced numbers of myelinating oligodendrocytes and hypomyelination due to decreased OPC proliferation rather than failed specification of the oligodendrocyte lineage. In addition, transient overexpression of gpr56 in wild-type (WT) zebrafish increases numbers of pro-oligodendrocytes but inhibits terminal differentiation of mature oligodendrocytes. Finally, we show that these functions are mediated by interactions with Gα 12/13 G-proteins and RhoA signalling. Together, our studies implicate Gpr56 as an essential regulator of oligodendrocyte development and myelination. gpr56 is expressed during oligodendrocyte development Myelin is an evolutionary innovation of the jawed vertebrate lineage [23] , and zebrafish represent one of the simplest genetically tractable organisms in which to study myelinating glial cell development. We therefore took advantage of the zebrafish model system to interrogate the necessity of Gpr56 function in oligodendrocyte development and myelination. First, we analysed the spatiotemporal expression of gpr56 by RT–PCR in developing zebrafish. We detected gpr56 expression during embryogenesis and in early larval stages (2 through 5 days post-fertilization (dpf)) when OPCs are first specified and differentiated [24] ( Fig. 1a ). In addition, whole-mount in situ hybridization (WISH) revealed low levels of gpr56 expression throughout the CNS at 1 dpf, before OPC specification [24] ( Fig. 1b ). These findings are consistent with previously published data in mammals showing that Gpr56 is also expressed in astrocytes, and to a lesser extent, in neurons [18] . At 2 dpf, when OPCs have been specified and are actively migrating and dividing [24] , there was a marked increase in gpr56 expression in the CNS ( Fig. 1c ). Cross-sections of 2 dpf WISH embryos revealed that gpr56 is expressed along the spinal cord midline and in a single distinct band running dorsal to ventral on either side of the midline, consistent with expression in neural precursors ( Fig. 1d ). In contrast, gpr56 expression was not detected by WISH in the CNS at larval stages >3 dpf ( Supplementary Fig. 1a,b ), during which time oligodendrocytes undergo terminal differentiation [24] , [25] . We also never detected signal in sense control WISH experiments ( Supplementary Fig. 1c ). These findings demonstrate that gpr56 expression during CNS development is conserved from zebrafish to mammals and suggest that levels are highest at earlier stages. 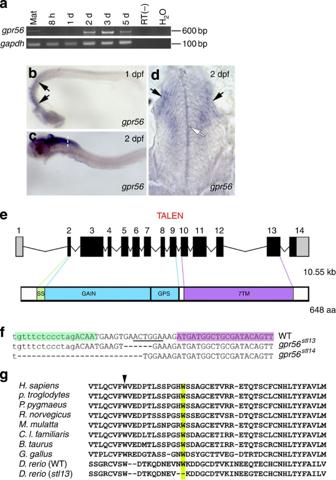Figure 1:gpr56expression and mutant generation in zebrafish. (a) Representative image ofgpr56expression assessed by RT–PCR from fertilization through larval development (three technical replicates). From left to right: Mat (maternal expression), 8 h (8 h post-fertilization), 1 d (days post-fertilization) to 5 d, RT (-) control and H20 control. (b,c) Whole-mountin situhybridization (WISH) of zebrafish larvae at (b) 1 and (c) 2 dpf shows robustgpr56expression within the central nervous system (black arrows inb) during larval development (lateral views shown, anterior to the left, dorsal is up, two technical replicates performed). (d) Cross-section through the spinal cord (white dashed line incdepicts approximate location) ofgpr56WISH embryo at 2 dpf showsgpr56expression in the spinal cord midline (white arrow) and in bands consistent with neural precursors (black arrows). (e) Diagram of the zebrafishgpr56gene (top) and protein (bottom) structures. TALENs used to generategpr56zebrafish mutants targeted between the 8th and 9th exons (text in red). Gpr56 contains a signal sequence (ss), GPCR Autoproteolysis-Inducing Domain (GAIN), GPCR Proteolytic Site (GPS) and the canonical 7-Transmembrane Domain (7TM). (f) Recovered mutant alleles ofgpr56—stl13representing a 6-bp deletion andstl14representing a 26 bp deletion. (g) Amino-acid sequence alignment of the GPS motif from representative species showing perfect conservation of the Trp residue that is deleted in thegpr56stl13/stl13allele (highlighted yellow). Mutation of the second, highly conserved Trp residue within the GPS causes BFPP (black arrowhead). Figure 1: gpr56 expression and mutant generation in zebrafish. ( a ) Representative image of gpr56 expression assessed by RT–PCR from fertilization through larval development (three technical replicates). From left to right: Mat (maternal expression), 8 h (8 h post-fertilization), 1 d (days post-fertilization) to 5 d, RT (-) control and H 2 0 control. ( b , c ) Whole-mount in situ hybridization (WISH) of zebrafish larvae at ( b ) 1 and ( c ) 2 dpf shows robust gpr56 expression within the central nervous system (black arrows in b ) during larval development (lateral views shown, anterior to the left, dorsal is up, two technical replicates performed). ( d ) Cross-section through the spinal cord (white dashed line in c depicts approximate location) of gpr56 WISH embryo at 2 dpf shows gpr56 expression in the spinal cord midline (white arrow) and in bands consistent with neural precursors (black arrows). ( e ) Diagram of the zebrafish gpr56 gene (top) and protein (bottom) structures. TALENs used to generate gpr56 zebrafish mutants targeted between the 8th and 9th exons (text in red). Gpr56 contains a signal sequence (ss), GPCR Autoproteolysis-Inducing Domain (GAIN), GPCR Proteolytic Site (GPS) and the canonical 7-Transmembrane Domain (7TM). ( f ) Recovered mutant alleles of gpr56 — stl13 representing a 6-bp deletion and stl14 representing a 26 bp deletion. ( g ) Amino-acid sequence alignment of the GPS motif from representative species showing perfect conservation of the Trp residue that is deleted in the gpr56 stl13/stl13 allele (highlighted yellow). Mutation of the second, highly conserved Trp residue within the GPS causes BFPP (black arrowhead). Full size image Targeted disruption of gpr56 in zebrafish Given the expression pattern of gpr56 in the developing CNS, we sought to test the hypothesis that Gpr56 regulates oligodendrocyte development. To this end, we generated Transcription Activator-Like Effector Nucleases (TALENs) [26] designed to cleave zebrafish gpr56 genomic sequences between exons 8 and 9 ( Fig. 1e ), which encode the GPS motif. We recovered two mutant alleles of gpr56: stl13 representing a 6 bp deletion that is predicted to remove a completely conserved tryptophan residue, and stl14 representing a 26 bp deletion ( Fig. 1f,g ). The GPS is a cysteine-rich domain containing four cysteine residues and two tryptophan residues required for autoproteolytic cleavage [27] . Previous reports show that inhibiting autoproteolytic cleavage of GPR56 prevents receptor trafficking and therefore impairs signalling [20] . In addition, two missense mutations that disrupt the highly conserved cysteine and tryptophan residues in humans cause BFPP [27] . Together, these findings suggest that gpr56 stl13/stl13 mutants may generate a non-functional Gpr56 due to failed trafficking of the receptor to the plasma membrane. Therefore, we chose to primarily characterize and utilize stl13 as a tool for understanding gpr56 function. Gpr56 is required for proper oligodendrocyte development To determine whether Gpr56 is required for normal oligodendrogliogenesis, we performed marker analyses to observe oligodendrocyte development in gpr56 stl13/stl13 mutants. In the CNS, OPCs differentiate from neural progenitors that reside within subventricular zones of the embryonic brain and spinal cord through coordinated expression of the transcription factors Olig2 and Sox10 (ref. 28 ). Some OPCs remain as non-myelinating OPC progenitors throughout life, while others are further specified by expression of the transcription factor Nkx2.2 , which allows OPCs to enter the terminal differentiation pathway. Expression of Nkx2.2 is characteristic of axon-associated pro-oligodendrocytes (pro-OLs) [25] , and mature myelinating oligodendrocytes express Myelin basic protein ( Mbp ), which encodes a structural component of the myelin sheath [28] . Using transgenic sox10(−7.2):memgfp zebrafish (a kind gift from M. Voigt, manuscript in preparation), we did not detect any difference in the number of sox10 + OPCs in gpr56 stl13/13 larvae ( N =19) compared with controls ( N =20) at 28 hours post-fertilization (hpf), the earliest time point at which sox10 expression was detected ( Fig. 2a–c , P <0.09, Student’s t -test). These data suggest that specification of the oligodendrocyte lineage is not impaired in gpr56 stl13/stl13 mutants. Consistent with this observation, general dorsal-ventral patterning (visualized by Sonic hedgehog pathway markers) was also unaffected in gpr56 stl13/13 mutants ( Supplementary Fig. 2 ). Furthermore, we did not observe overt defects in the development of neurons, radial glia, or in microglia number at any stage examined in gpr56 stl13/13 mutants compared with controls ( Supplementary Fig. 3 ). However, by 2.5 dpf, we detected a significant decrease ( P < 5.223x10 −6 , Student’s t -test) in nkx2.2a + pro-OL number in gpr56 stl13/13 mutants ( N =19) by WISH relative to controls ( gpr56 +/+ and gpr56 stl13/+ : N =22), and we observed a subsequent reduction in CNS mbp expression in gpr56 mutants ( gpr56 stl13/stl13 : N =20/27 , gpr56 stl14/stl14 : N =14/19) by 4 dpf ( Fig. 2d–i , WT control: N =13/13). Although gpr56 is maternally expressed ( Fig. 1a ), we did not observe enhanced defects in oligodendrocyte development in gpr56 stl13/stl13 maternal-zygotic mutants (no WT maternal contribution) compared with gpr56 stl13/stl13 zygotic mutants ( Fig. 2j , N =5/5). Importantly, injection of synthetic mRNA encoding WT zebrafish (50 pg) or mouse (200 pg) Gpr56 was sufficient to rescue the CNS mbp deficits in gpr56 stl13/stl13 mutants, confirming the specificity of the TALEN-induced mutations ( Supplementary Fig. 4 ). Together, these results demonstrate that Gpr56 is required for the proper development of mature, myelinating oligodendrocytes. 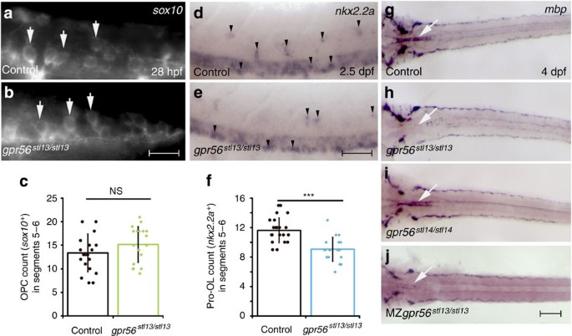Figure 2: Oligodendrocyte development is impaired ingpr56zebrafish mutants. (a,b) Representative fluorescent images of (a) control (gpr56stl13/+) and (b)gpr56stl13/13larvae at 28 hpf expressingTg(sox10(−7.2):memGFP)to mark OPCs. (c) Quantification of OPC number (sox10+; white arrows) in control (N=20) andgpr56stl13/stl13(N=19) larvae. (d–f) Representative WISH images of the spinal cord of (e)gpr56stl13/stl13(N=19) and (d) control embryos (gpr56+/+andgpr56stl13/+,N=22) showingnkx2.2aexpression to mark pro-OLs. (f) Quantification of pro-OL number (nkx2.2a+) (P<5.223 × 10−6). (g–j)mbpexpression (CNS marked by white arrow, hindbrain) in (h)gpr56stl13/13(N=20/27), (i)gpr56stl14/stl14(N=14/19) and (j) MZgpr56stl/13/stl13(5/5) larvae compared with (g) WT controls at 4 dpf (N=13/13). (a–f) All images and quantification thereof were taken from segments 5 to 6 for consistency. For (a,b,d,e) lateral views are shown, anterior to the left, dorsal is up; for (g–j) dorsal views are shown, anterior to the left. (a,b) Scale bar, 50 μm. (d,e) Scale bar, 100 μm. (g–j) Scale bar, 200 μm. Student’st-test used to test for statistical significance and error bars shown as±s.d. A minimum of two technical replicates were performed for each marker. NS, not significant. Figure 2: Oligodendrocyte development is impaired in gpr56 zebrafish mutants. ( a , b ) Representative fluorescent images of ( a ) control ( gpr56 stl13/+ ) and ( b ) gpr56 stl13/13 larvae at 28 hpf expressing Tg(sox10(−7.2):memGFP) to mark OPCs. ( c ) Quantification of OPC number ( sox10+ ; white arrows) in control ( N =20) and gpr56 stl13/stl13 ( N= 19) larvae. ( d – f ) Representative WISH images of the spinal cord of ( e ) gpr56 stl13/stl13 ( N =19) and ( d ) control embryos ( gpr56 +/+ and gpr56 stl13/+ , N =22) showing nkx2.2a expression to mark pro-OLs. ( f ) Quantification of pro-OL number ( nkx2.2a +) ( P <5.223 × 10 −6 ). ( g – j ) mbp expression (CNS marked by white arrow, hindbrain) in ( h ) gpr56 stl13/13 ( N =20/27), ( i ) gpr56 stl14/stl14 ( N =14/19) and ( j ) MZ gpr56 stl/13/stl13 (5/5) larvae compared with ( g ) WT controls at 4 dpf ( N =13/13). ( a – f ) All images and quantification thereof were taken from segments 5 to 6 for consistency. For ( a , b , d , e ) lateral views are shown, anterior to the left, dorsal is up; for ( g – j ) dorsal views are shown, anterior to the left. ( a , b ) Scale bar, 50 μm. ( d , e ) Scale bar, 100 μm. ( g – j ) Scale bar, 200 μm. Student’s t -test used to test for statistical significance and error bars shown as±s.d. A minimum of two technical replicates were performed for each marker. NS, not significant. Full size image Mutations in gpr56 cause CNS hypomyelination To further delineate how impaired Gpr56 function affects oligodendrocyte myelination, we performed transmission electron microscopy (TEM) to measure the extent and quality of myelin present in the ventral spinal cord of gpr56 mutants ( gpr56 stl13/stl13 : N =5 , gpr56 stl14/stl14 : N =4, WT: N =6) during development ( Fig. 3a–k ). We found a significant reduction ( gpr56 stl13/stl13 , P <0.019 ; gpr56 stl14/stl14 , P <0.039, Student’s t -test) in the percent of myelinated axons in mutant larvae compared with WT controls at 5 dpf ( Fig. 3l ), but total axon number was unchanged ( gpr56 stl13/stl13 , P <0.5 ; gpr56 stl14/stl14 , P <0.78, Student’s t -test Fig. 3m ). We also did not observe a change in the number of myelin wraps surrounding those axons that were myelinated in gpr56 stl13/stl13 mutants compared with controls ( Fig. 3n,o ; non-Mauthner: gpr56 stl13/stl13 : P <0.29, gpr56 stl14/stl14 : P <0.6; Mauthner: gpr56 stl13/stl13 : P <0.25, gpr56 stl14/stl14 : P <0.76, Student’s t -test). In contrast to the hypomyelination phenotype shown in the ventral spinal cord of gpr56 mutants at 5 dpf ( Fig. 3f–k ), we did not observe any effect on oligodendrocyte myelination in the dorsal spinal cord at this developmental stage ( Supplementary Fig. 5 ). By 21 dpf, however, we observed a statistically significant decrease in the percent of myelinated axons in the ventral ( P <0.007, Student’s t -test) and dorsal ( P <0.002) spinal cord of gpr56 stl13/stl13 ( N =4) mutants relative to WT siblings ( N =2), with no change in axon number ( Supplementary Fig. 6 , dorsal spinal cord: P <0.89, ventral spinal cord: P <0.96, Student’s t -test). We suspect that we were unable to detect a difference in the dorsal spinal cord at larval stages because very few axons are myelinated in this region at 5 dpf. Interestingly, we also observed many oligodendrocytes with distended endoplasmic reticulum in gpr56 stl13/stl13 mutants at 21 dpf, which was rarely seen in controls, supporting the hypothesis that the protein encoded by gpr56 stl13/stl13 does not traffic properly from the endoplasmic reticulum to the plasma membrane ( Supplementary Fig. 6 ). To determine if myelination is simply delayed in gpr56 stl13/stl13 mutants, we analysed myelin ultrastructure in the spinal cord of gpr56 stl13/stl13 animals at 6 months of age ( Supplementary Fig. 7 ). At 6 months, we likewise found a statistically significant decrease in the percent of myelinated axons in gpr56 stl13/stl13 mutants ( N =4) compared with WT controls ( N =3) in both the ventral ( Supplementary Fig. 7g , axon diameter of 0.2–0.5 μm ( P <0.021), 0.5–1 μm ( P <0.005) and 1–2 μm ( P <0.029), Student’s t -test) and dorsal spinal cord ( Supplementary Fig. 7n , axon diameter of 0.2–0.5 μm ( P <0.003) and 0.5–1 μm ( P <0.008), Student’s t -test), without any change in myelin thickness for axons that were myelinated ( Supplementary Fig. 7h,o , linear regression analysis). Axon number was also unchanged in mutants compared with controls ( Supplementary Fig. 7f,m , dorsal spinal cord: P <0.11, ventral spinal cord: P <0.34, Student’s t -test). Collectively, our analysis demonstrates that altered Gpr56 function causes developmental CNS hypomyelination that persists in the adult spinal cord. 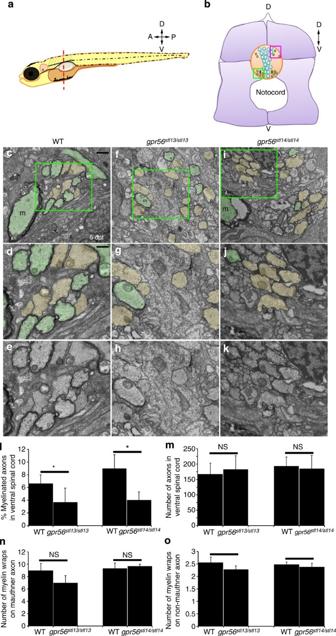Figure 3:gpr56mutant spinal cord axons are hypomyelinated. (a) Schematic representation of a 5 dpf zebrafish. Larvae were cut between segments 5 and 6 (red dashed line) and prepared for TEM. Axis shows orientation of the embryo (D, dorsal; V, ventral; A, anterior; P, posterior). (b) Diagram of a 5 dpf zebrafish cross-section, dorsal is up (D), ventral is down (V). In this image, the spinal cord is in orange and includes neuronal cell bodies (blue) and myelinated axons (green). Ventral region used for quantification is boxed in green, dorsal region used for quantification boxed in magenta. Muscle in purple. (c–k) Representative TEM images from the ventral spinal cord of WT (c–e,N=6),gpr56stl13/stl13mutant larvae (f–h,N=5), andgpr56stl14/stl14mutant larvae (i–k,N=4) at 5 dpf. Higher magnifications ofc,f,iare shown ind–e,g–h,j–k, respectively. (c,d,f,g,i,j) Myelinated axons are shaded green, unmyelinated large caliber axons (≥ 500 nm) are shaded orange. (e,h,k) Images from panelsd,g,jwithout pseudocolour. (l) Quantification of the percent of myelinated axons in the ventral spinal cord ofgpr56stl13/stl13(P<0.019) andgpr56stl14/stl14(P<0.039) compared with WT controls. (m) Quantification of the total number of axons in the ventral spinal cord ofgpr56stl13/stl13(P<0.5) andgpr56stl14/stl14(P<0.78) compared with WT controls. (n,o) We also did not observe a significant difference in the number of myelin wraps per myelinated axon in mutants compared with control on the large caliber Mauthner axon (m) or on smaller caliber myelinated axons. (c,f,i) Scale bar, 1 μm. (d,e,g,h,j,k) Scale bar, 500 nm. (l–o) Quantification performed on a stereotyped 14 μm2region (b) in the ventral spinal cord. Student’st-test used to test for statistical significance and error bars shown as±s.d. NS, not significant. Data represent two technical replicates. Figure 3: gpr56 mutant spinal cord axons are hypomyelinated. ( a ) Schematic representation of a 5 dpf zebrafish. Larvae were cut between segments 5 and 6 (red dashed line) and prepared for TEM. Axis shows orientation of the embryo (D, dorsal; V, ventral; A, anterior; P, posterior). ( b ) Diagram of a 5 dpf zebrafish cross-section, dorsal is up (D), ventral is down (V). In this image, the spinal cord is in orange and includes neuronal cell bodies (blue) and myelinated axons (green). Ventral region used for quantification is boxed in green, dorsal region used for quantification boxed in magenta. Muscle in purple. ( c – k ) Representative TEM images from the ventral spinal cord of WT ( c – e , N =6), gpr56 stl13/stl13 mutant larvae ( f – h , N =5), and gpr56 stl14/stl14 mutant larvae ( i – k , N =4) at 5 dpf. Higher magnifications of c , f , i are shown in d – e , g – h , j – k , respectively. ( c , d , f , g , i , j ) Myelinated axons are shaded green, unmyelinated large caliber axons (≥ 500 nm) are shaded orange. ( e , h , k ) Images from panels d , g , j without pseudocolour. ( l ) Quantification of the percent of myelinated axons in the ventral spinal cord of gpr56 stl13/stl13 ( P <0.019) and gpr56 stl14/stl14 ( P <0.039) compared with WT controls. ( m ) Quantification of the total number of axons in the ventral spinal cord of gpr56 stl13/stl13 ( P <0.5) and gpr56 stl14/stl14 ( P <0.78) compared with WT controls. ( n , o ) We also did not observe a significant difference in the number of myelin wraps per myelinated axon in mutants compared with control on the large caliber Mauthner axon (m) or on smaller caliber myelinated axons. ( c , f , i ) Scale bar, 1 μm. ( d , e , g , h , j , k ) Scale bar, 500 nm. ( l – o ) Quantification performed on a stereotyped 14 μm 2 region ( b ) in the ventral spinal cord. Student’s t -test used to test for statistical significance and error bars shown as±s.d. NS, not significant. Data represent two technical replicates. Full size image Gpr56 is not required for neural stem cell differentiation One possible explanation for the observed decrease in myelinating oligodendrocyte numbers in gpr56 stl13/stl13 mutants could be reduced differentiation of the oligodendrocyte lineage from neural stem cells. The fact that we did not detect defects in early OPC specification ( Fig. 2a–c ) in gpr56 stl13/stl13 zebrafish mutants argued against this, but, to definitively test this model, we harvested neurospheres from the subventricular zone of Gpr56 −/− knockout mice [29] at postnatal day 3 and assessed their ability to differentiate into Tuj1+ neurons, GFAP+ astrocytes and O4+ oligodendrocytes. Importantly, we found robust levels of the Gpr56 protein in neurospheres harvested from WT and Gpr56 +/− animals, which was absent from mutant neurospheres ( Supplementary Fig. 8 ). We observed no differences in the ability of Gpr56 −/− neural stem cells to differentiate into any cell-type tested ( Fig. 4 ), consistent with our analysis of gpr56 stl13/stl13 zebrafish mutants ( Fig. 2a–c ; Supplementary Fig. 3 ). Of note, neurospheres harvested from the spinal cord of Gpr56−/− animals showed a slightly increased potential to differentiate into neurons ( Supplementary Fig. 9 ), highlighting the variation that exists between neural progenitor populations from different tissues [30] . Importantly, neurospheres harvested from both tissues showed no difference in their ability to differentiate into oligodendrocytes compared with controls, supporting the hypothesis that Gpr56 is not required for specification and differentiation of the oligodendrocyte lineage. 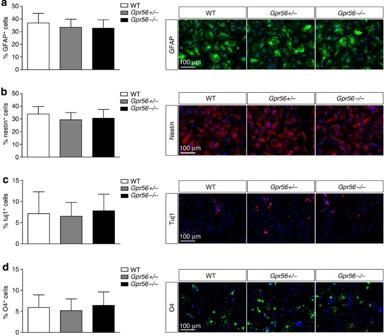Figure 4: Loss ofGpr56does not affect neural precursor differentiation capacity. Quantification of the percent of (a) GFAP+ astrocytes, (b) Nestin+ neural progenitors, (c) Tuj1+ neurons and (d) O4+ oligodendrocytes (per field of view) differentiated from neural precursors harvested from WT (N=3),Gpr56+/−(N=4), andGpr56−/−(N=5) animals at postnatal day 3 (P3). Representative fluorescent images from each genotype shown to the right of each summary graph. Two-way ANOVA used to test for statistical significance and error bars shown as±s.d. Data were acquired from two technical replicates. Figure 4: Loss of Gpr56 does not affect neural precursor differentiation capacity. Quantification of the percent of ( a ) GFAP+ astrocytes, ( b ) Nestin+ neural progenitors, ( c ) Tuj1+ neurons and ( d ) O4+ oligodendrocytes (per field of view) differentiated from neural precursors harvested from WT ( N =3), Gpr56+/− ( N =4), and Gpr56−/− ( N =5) animals at postnatal day 3 (P3). Representative fluorescent images from each genotype shown to the right of each summary graph. Two-way ANOVA used to test for statistical significance and error bars shown as±s.d. Data were acquired from two technical replicates. Full size image Gpr56 regulates OPC proliferation Because OPC specification is unaffected in gpr56 stl13/stl13 zebrafish mutants, and loss of Gpr56 does not affect the ability of neural precursors to differentiate into oligodendrocytes, reduced pro-OL numbers in gpr56 stl13/stl13 mutants could result from increased death and/or decreased proliferation of OPCs. To distinguish between these possibilities, we performed time-lapse imaging of gpr56 stl13/stl13 mutants and controls using transgenic sox10(−7.2):mRFP [24] zebrafish to visualize OPC behaviour and development in vivo ( Supplementary Movies 1 and 2 ). Embryos were imaged from 30 to 46 hpf, allowing us to monitor the transition of many OPCs into pro-OLs. At 30 hpf, we found a statistically significant increase in the number of axons associated with pro-OLs in gpr56 stl13/stl13 mutants ( N =7) compared with controls ( N =7 , P <0.04, Student’s t -test). Over time, however, the number of pro-OL associated axons in control embryos increased at a higher rate than in gpr56 stl13/stl13 mutants. This increase resulted in a statistically significant reduction in pro-OL associated axons in gpr56 stl13/stl13 mutants compared with controls by 46 hpf ( Fig. 5a–c , P <0.004, Student’s t -test), consistent with our marker analysis ( Fig. 2d–f ). These findings suggest that in gpr56 stl13/stl13 mutants, OPCs are born and prematurely form associations with axons, but that they do not proliferate sufficiently to account for the total number of axons that need to be myelinated. In accordance with this hypothesis, we also observed additional myelinated axons in the ventral spinal cord of gpr56 stl13/stl13 mutants ( N =3) compared with controls (WT: N =3 , gpr56 stl13/+− : N =3) by TEM at 3 dpf ( Fig. 5d–g , P <0.048, Student’s t -test), indicative of precocious myelination. In addition, we observed a statistically significant reduction in the number of proliferating OPCs ( sox10+; pH3+) in gpr56 stl13/stl13 mutants compared with controls at 32 hpf, when most OPCs have not yet entered the differentiation programme [24] , [25] ( Fig. 5h–j , P <0.0004, Student’s t -test). Importantly, we did not observe any signs of cell death via time-lapse imaging, and there was no increase in the number of cell corpses assessed by acridine orange staining at 32 hpf, 2 dpf or 3 dpf in gpr56 stl13/stl13 mutants compared with controls ( Fig. 5k–m ). Thus, changes in pro-OL number can only be attributed to changes in OPC proliferation and not cell death. Together, these data support a model in which Gpr56 promotes OPC proliferation at the expense of differentiation such that, when Gpr56 function is impaired, insufficient OPC proliferation results in fewer pro-OLs and mature oligodendrocytes, which leads to hypomyelination. 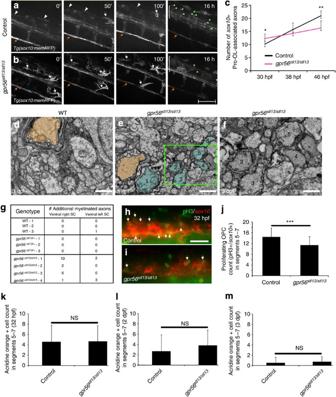Figure 5:gpr56mutant OPCs form premature associations with axons and are less proliferative than controls. (a,b) Representative stills fromin vivotime-lapse imaging of the spinal cord (white bracket at 16 h) from segments 5 to 7 of (a) controls (gpr56stl13/+,N=6) and (b)gpr56stl13/stl13mutants (N=7) expressingtg(sox10(−7.2):mRFP) to visualize OPC behaviour over time (three technical replicates performed). Embryos were imaged from 30 to 46 hpf to encompass the transition of OPCs (white arrowheads) into pro-OLs (light green arrowheads). White arrows denotesox10expressing neural crest cells, and orange arrows mark the posterior lateral line nerve, which is part of the peripheral nervous system and is marked by the presence of migrating Schwann cell precursors. (c) Quantification of the number of pro-OL associated axons over time ingpr56mutants compared with controls at 30 hpf (P<0.039), 38 hpf (P<0.28) and 46 hpf (P=0.004). (d–f) Representative TEM images of the ventral spinal cord of a WT (d,N=3) andgpr56stl13/stl13(e,f,N=4) embryo at 3 dpf (two technical replicates performed). (e) Additional non-Mauthner myelinated axons (shaded blue and numbered) were observed ingpr56stl13/stl13embryos (P<0.048) compared with controls. Mauthner axon shaded orange. (f) Image shows a higher magnification of panele(green box). (g) Raw counts of non-Mauthner myelinated axons in control andgpr56stl13/stl13embryos at 3 dpf. (h,i) Representative fluorescent images of the spinal cord from segments 5 to 7 of (h) control (gpr56stl13/+,N=31) and (i)gpr56stl13/stl13mutant (N=34) embryos at 32 hpf (two technical replicates performed). Embryos expressingtg(sox10 (−7.2):mRFP) were fixed and stained with pH3 to assay proliferation. (j) Quantification of the number of proliferating OPCs ingpr56stl13/stl13mutants compared with controls (P<0.0004). (k–m) Quantification of dying cells (acridine orange +, one technical replicate per time point) ingpr56stl13/stl13mutants and controls (WT andgpr56stl13/+) at 32 hpf (control:N=13, gpr56stl13/stl13:N=20), 2 dpf (control:N=21, gpr56stl13/stl13:N=12) and 3 dpf (control:N=19, gpr56stl13/stl13:N=20). (a,b,h,i) Scale bar, 50 μm. (d,e) Scale bar, 1 μm. (f) Scale bar, 500 nm. Student’st-test used to test for statistical significance and error bars shown as±s.d. Figure 5: gpr56 mutant OPCs form premature associations with axons and are less proliferative than controls. ( a , b ) Representative stills from in vivo time-lapse imaging of the spinal cord (white bracket at 16 h) from segments 5 to 7 of ( a ) controls ( gpr56 stl13/+ , N =6) and ( b ) gpr56 stl13/stl13 mutants ( N =7) expressing tg(sox10(−7.2):mRFP ) to visualize OPC behaviour over time (three technical replicates performed). Embryos were imaged from 30 to 46 hpf to encompass the transition of OPCs (white arrowheads) into pro-OLs (light green arrowheads). White arrows denote sox10 expressing neural crest cells, and orange arrows mark the posterior lateral line nerve, which is part of the peripheral nervous system and is marked by the presence of migrating Schwann cell precursors. ( c ) Quantification of the number of pro-OL associated axons over time in gpr56 mutants compared with controls at 30 hpf ( P <0.039), 38 hpf ( P <0.28) and 46 hpf ( P =0.004). ( d – f ) Representative TEM images of the ventral spinal cord of a WT ( d , N =3) and gpr56 stl13/stl13 ( e , f , N =4) embryo at 3 dpf (two technical replicates performed). ( e ) Additional non-Mauthner myelinated axons (shaded blue and numbered) were observed in gpr56 stl13/stl13 embryos ( P <0.048) compared with controls. Mauthner axon shaded orange. ( f ) Image shows a higher magnification of panel e (green box). ( g ) Raw counts of non-Mauthner myelinated axons in control and gpr56 stl13/stl13 embryos at 3 dpf. ( h , i ) Representative fluorescent images of the spinal cord from segments 5 to 7 of ( h ) control ( gpr56 stl13/+ , N =31) and ( i ) gpr56 stl13/stl13 mutant ( N =34) embryos at 32 hpf (two technical replicates performed). Embryos expressing tg(sox10 (−7.2):mRFP ) were fixed and stained with pH3 to assay proliferation. ( j ) Quantification of the number of proliferating OPCs in gpr56 stl13/stl13 mutants compared with controls ( P <0.0004). ( k – m ) Quantification of dying cells (acridine orange +, one technical replicate per time point) in gpr56 stl13/stl13 mutants and controls (WT and gpr56 stl13/+ ) at 32 hpf (control: N =13 , gpr56 stl13/stl13 : N =20), 2 dpf (control: N =21 , gpr56 stl13/stl13 : N =12) and 3 dpf (control: N =19 , gpr56 stl13/stl13 : N =20). ( a , b , h , i ) Scale bar, 50 μm. ( d , e ) Scale bar, 1 μm. ( f ) Scale bar, 500 nm. Student’s t -test used to test for statistical significance and error bars shown as±s.d. Full size image gpr56 OE increases OPC number but inhibits myelination Impaired Gpr56 function results in reduced numbers of myelinating oligodendrocytes and myelin due to decreased OPC proliferation ( Figs 2 , 3 and 5 , Supplementary Figs 6 and 7 ). Transient overexpression (OE) of WT Gpr56 synthetic mRNA rescues CNS mbp expression ( Supplementary Fig. 4 ) by suppressing the OPC proliferation defect observed in gpr56 stl13/stl13 mutants ( Supplementary Fig. 10 ). Interestingly, we also observed enhanced mbp expression in a large fraction of gpr56 -injected embryos ( Supplementary Fig. 4d,e ). We therefore hypothesized that transient OE of gpr56 in WT embryos would cause hypermyelination by increasing oligodendrocyte number. Analysis of nkx2.2a expression revealed a statistically significant increase in the number of nkx2.2a + pro-OLs in the anterior ( P < 8.7x10 −7 , Student’s t -test) and posterior ( P <0.01, Student’s t -test) spinal cord ( Fig. 6a–f ) of embryos injected with 50 pg of WT gpr56 synthetic mRNA (anterior: N =25, posterior: N =29) relative to control-injected embryos (anterior: N =26, posterior: N =31). In addition, we noted an increase in CNS mbp expression in gpr56 -OE embryos relative to phenol-red-injected controls by WISH ( Fig. 6g–j , N=19/34) at 2.5 dpf. Consistent with these findings, we observed an increase in the numbers of oligodendrocyte lineage nuclei in the spinal cord of gpr56 -OE embryos relative to phenol-red-injected controls by TEM at 2.5 and 5 dpf ( Fig. 6l–q ; P <0.037 at 2.5 dpf (OE: N =4, control-injected: N =4); P <0.15 at 5 dpf (OE: N =5, control-injected: N =4), Student’s t -test). We distinguished oligodendrocyte and OPC nuclei from neuronal nuclei by their distinctive heterochromatin conformations. OPC and oligodendrocyte heterochromatin is heavily condensed and localized along the perimeter of the nucleus for OPCs or in patches throughout for post-mitotic, terminally differentiated oligodendrocytes. In contrast, neuronal heterochromatin is organized uniformly throughout the nucleus, often with a single dense nucleolus [31] , [32] , [33] . At 2.5 dpf, generally only the large Mauthner axons are myelinated in WT zebrafish [34] , but, in some OE embryos, additional myelinated axons were observed compared with controls at this time point by TEM ( N =2/4 in the ventral spinal cord and N =1/4 in the dorsal spinal cord, Supplementary Fig. 11 ), although the difference was not significant. Taken alone, these data suggest that OE of gpr56 may induce hypermyelination; however, we observed hypomyelination in gpr56 OE embryos relative to controls at 5 dpf by TEM ( Fig. 6r–x ). These findings indicate that OE of gpr56 increases mbp expression by increasing pro-OL number but that this mbp expression is not equivalent to true myelination, and OE of gpr56 inhibits terminal differentiation and myelination. Collectively, these data support the hypothesis that Gpr56 is both a positive regulator of OPC proliferation and a negative regulator of oligodendrocyte differentiation. 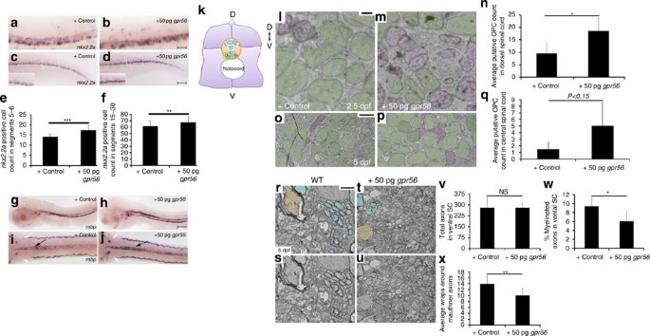Figure 6: Overexpression ofgpr56causes increased OPC number and inhibits myelination. (a–d) WISH showsnkx2.2aexpression in the spinal cord of injected WT larvae at 2.5 dpf. Lateral views are shown, dorsal is up. (e,f) Quantification of the number ofnkx2.2a+ pro-OLs (black arrowheads) in WT embryos injected with 50 pg of syntheticgpr56mRNA (N=30) in the anterior (b, segments 5–6,P<8.7 × 10−7) and posterior (d, segments 15–30,P<0.01) spinal cord compared with injected controls (a,c,N=31). (g–j) Representative images of a (h,j)gpr56-injected WT larva (N=19/31) compared with a (g,i) control-injected embryo (N=33/35) showingmbpexpression by WISH. (g,h) Lateral views shown, anterior on right. (i,j) Dorsal views shown, anterior on right. Black arrows. (k) Cartoon of zebrafish larva in cross-section modified fromFig. 3b. White box represents regions shown inl,m,o,p. Green box represents region shown inr–u. (l,m,o,p) Representative images of spinal cord cross-sections from 2.5 dpf (l,m) and 5 dpf (o,p) WT embryos injected with control (l,o) or 50 pggpr56synthetic mRNA (m,p). 2.5 dpf: scale bar, 500 nm. 5 dpf: scale bar, 4 μm. (n,q) Quantification of the number of oligodendrocyte lineage cell bodies (shaded purple) ingpr56-injected embryos (N=4) compared with controls (N=4) at 2.5 dpf (P<0.037) and 5 dpf (P<0.15,N=4 for controls andN=5 forgpr56-injected embryos). Neuronal cell bodies shaded green. (r–u) Representative TEM images of the spinal cord in cross-section from 5 dpf control (r,s) andgpr56-injected (t,u) embryos. Scale bar, 1 μm. Quantification of total axon number (v), % myelinated axons (shaded blue,w,P<0.05) and myelin thickness on the large caliber Mauthner axon (shaded orange,x,P<0.008) ingpr56OE embryos at 5 dpf relative to controls. SC, spinal cord. Student’st-test used to test for statistical significance and error bars shown as±s.d. Two technical replicates were performed for each overexpression experiment. Figure 6: Overexpression of gpr56 causes increased OPC number and inhibits myelination. ( a – d ) WISH shows nkx2.2a expression in the spinal cord of injected WT larvae at 2.5 dpf. Lateral views are shown, dorsal is up. ( e , f ) Quantification of the number of nkx2.2a + pro-OLs (black arrowheads) in WT embryos injected with 50 pg of synthetic gpr56 mRNA ( N =30) in the anterior ( b , segments 5–6, P <8.7 × 10 −7 ) and posterior ( d , segments 15–30, P <0.01) spinal cord compared with injected controls ( a , c , N =31). ( g – j ) Representative images of a ( h , j ) gpr56 -injected WT larva ( N =19/31) compared with a ( g , i ) control-injected embryo ( N =33/35) showing mbp expression by WISH. ( g , h ) Lateral views shown, anterior on right. ( i , j ) Dorsal views shown, anterior on right. Black arrows. ( k ) Cartoon of zebrafish larva in cross-section modified from Fig. 3b . White box represents regions shown in l , m , o , p . Green box represents region shown in r – u . ( l , m , o , p ) Representative images of spinal cord cross-sections from 2.5 dpf ( l , m ) and 5 dpf ( o , p ) WT embryos injected with control ( l , o ) or 50 pg gpr56 synthetic mRNA ( m , p ). 2.5 dpf: scale bar, 500 nm. 5 dpf: scale bar, 4 μm. ( n , q ) Quantification of the number of oligodendrocyte lineage cell bodies (shaded purple) in gpr56 -injected embryos ( N =4) compared with controls ( N =4) at 2.5 dpf ( P <0.037) and 5 dpf ( P <0.15, N =4 for controls and N =5 for gpr56 -injected embryos). Neuronal cell bodies shaded green. ( r – u ) Representative TEM images of the spinal cord in cross-section from 5 dpf control ( r , s ) and gpr56 -injected ( t , u ) embryos. Scale bar, 1 μm. Quantification of total axon number ( v ), % myelinated axons (shaded blue, w , P <0. 05 ) and myelin thickness on the large caliber Mauthner axon (shaded orange, x , P <0.008) in gpr56 OE embryos at 5 dpf relative to controls. SC, spinal cord. Student’s t -test used to test for statistical significance and error bars shown as±s.d. Two technical replicates were performed for each overexpression experiment. Full size image Gα 12/13 and RhoA manipulations alter gpr56 mutant phenotypes Previous in vitro studies show that Gpr56 couples to Gα 12/13 and activates RhoA to control migration of mammalian neural precursor cells [35] , [36] . We likewise found that RhoA activity levels are high in control neurospheres when Gpr56 is abundant ( Supplementary Fig. 12 ). In OPCs, RhoA is highly expressed, but is later downregulated to facilitate terminal differentiation of oligodendrocytes in mammals [37] , which is consistent with the spatiotemporal expression profile we observe for gpr56 in zebrafish ( Fig. 1a–d ). Taken together, these data suggest that Gpr56 may couple to Gα 12/13 and activate RhoA during oligodendrocyte development. To test these hypotheses, we first used established antisense morpholino oligonucleotides that transiently impair Gα 12/13 function in gpr56 stl13/stl13 mutants through translational inhibition of three previously identified Gα 12/13 transcripts (‘3MO’; gna12 , gna13a and gna13b ) [38] . We then analysed mbp expression by WISH to assess oligodendrocyte development, and embryos were scored from 0 to 3 based on the strength of their expression: 0=nearly absent, 1=strongly reduced, 2=reduced, 3=wild type ( Fig. 7a–d ). We treated embryos with low doses of 3MO (1 ng each) such that WT, 3MO-injected embryos showed no phenotype ( Fig. 7e,f ). In contrast, sub-threshold doses of 3MO caused significant hypomyelination in gpr56 stl13/+ heterozygotes and severe hypomyelination in homozygous mutants, resulting in a marked shift in the distribution of their phenotypic classes and a significant reduction in their CNS mbp score ( Fig. 7e,f , control WT ( N =23) versus control heterozygote ( N =56): P <0.077; control WT ( N =23) versus control mutant ( N =32): P <0.0003; 3MO-injected WT ( N =10) versus 3MO-injected heterozygote ( N =36): P < 1.33x10 −5 ; 3MO-injected WT ( N =10) versus 3MO-injected mutant ( N =15): P < 2.59x10 −6 , Student’s t -test). As inhibition of Gα 12/13 function preferentially affects oligodendrocyte development in gpr56 stl13/+ heterozygotes and mutants compared with WT controls, our findings suggest a genetic interaction and thus support the hypothesis that Gpr56 promotes oligodendrocyte development via interactions with Gα 12/13 . 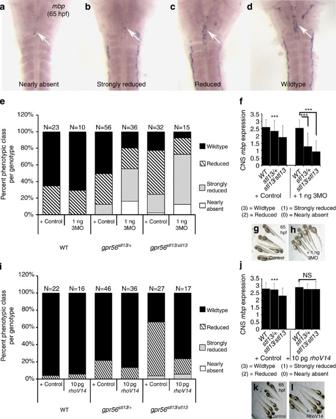Figure 7: Manipulation of Gα12/13and RhoA signalling influences CNSmbpexpression ingpr56mutants. (a–d) Injection of morpholinos (3MO) targeting Gα12/13signalling (gna12-MO,gna13a-MO andgna13b-MO, 1 ng each), constitutively activerhoasynthetic mRNA (10 pg), or phenol-red control yielded embryos with (d) WT, (c) reduced, (b) strongly reduced or (a) nearly absent CNSmbpexpression at 65 hpf by WISH (dorsal view shown, anterior is up, white arrows denote CNSmbpexpression). We scoredmbpexpression as follows: 3=WT, 2=reduced, 1=strongly reduced, 0=nearly absent. (e) Phenotypic distribution by genotype and treatment (1 ng 3MO or control-injected). (f) Quantification of CNSmbpscore by genotype and treatment (1 ng 3 MO or control-injected). (f) RespectivePvalues: control WT versus control heterozygote:P<0.077; control WT versus control mutant:P<0.0004; 3MO-injected WT versus 3MO-injected heterozygote:P<1.33 × 10−05; 3MO-injected WT versus 3MO-injected mutant:P<2.59 × 10−6). (i) Phenotypic distribution by genotype and treatment (10 pg consitutively active RhoA (rhoV14) or control-injected) (j) Quantification of CNSmbpscore by genotype and treatment (10 pg consitutively active RhoA (rhoV14) or control-injected). RespectiveP-values: control WT versus control mutant:P<0.0009; OE WT versus OE mutant:P<0.343. (g,h,k,l) All analysed injected embryos were morphologically normal. Student’st-test used to test for statistical significance and error bars are shown as±s.d. Two technical replicates were performed for the 3MO and the OE experiment. NS, not significant. Figure 7: Manipulation of Gα 12/13 and RhoA signalling influences CNS mbp expression in gpr56 mutants. ( a – d ) Injection of morpholinos (3MO) targeting Gα 12/13 signalling ( gna12 -MO, gna13a -MO and gna13b -MO, 1 ng each), constitutively active rhoa synthetic mRNA (10 pg), or phenol-red control yielded embryos with ( d ) WT, ( c ) reduced, ( b ) strongly reduced or ( a ) nearly absent CNS mbp expression at 65 hpf by WISH (dorsal view shown, anterior is up, white arrows denote CNS mbp expression). We scored mbp expression as follows: 3=WT, 2=reduced, 1=strongly reduced, 0=nearly absent. ( e ) Phenotypic distribution by genotype and treatment (1 ng 3MO or control-injected). ( f ) Quantification of CNS mbp score by genotype and treatment (1 ng 3 MO or control-injected). ( f ) Respective P values: control WT versus control heterozygote: P <0.077; control WT versus control mutant: P <0.0004; 3MO-injected WT versus 3MO-injected heterozygote: P <1.33 × 10 −05 ; 3MO-injected WT versus 3MO-injected mutant: P <2.59 × 10 −6 ). ( i ) Phenotypic distribution by genotype and treatment (10 pg consitutively active RhoA ( rhoV14 ) or control-injected) ( j ) Quantification of CNS mbp score by genotype and treatment (10 pg consitutively active RhoA ( rhoV14 ) or control-injected). Respective P -values: control WT versus control mutant: P <0.0009; OE WT versus OE mutant: P <0.343. ( g , h , k , l ) All analysed injected embryos were morphologically normal. Student’s t -test used to test for statistical significance and error bars are shown as±s.d. Two technical replicates were performed for the 3MO and the OE experiment. NS, not significant. Full size image Rho is the main downstream effector of Gα 12/13 (ref. 39 ), and previous studies in vitro implicate RhoA signalling downstream of Gpr56 (refs 35 , 36 ). We therefore hypothesized that Gpr56 couples to Gα 12/13 and signals through RhoA to promote oligodendrocyte development. Consistent with this model, transient OE of 10 pg of a constitutively active form of rhoa ( rhoV14 ) [38] suppressed gpr56 stl13/stl13 mutant phenotypes, including the OPC proliferation defect ( Supplementary Fig. 10 ) and CNS mbp score ( Fig. 7i,j , control WT ( N =22) versus control mutant ( N =27): P <0.0009; OE WT ( N =16) versus OE mutant ( N =17): P <0. 343 , Student’s t -test). OE of rhoa also caused a marked shift in the distribution of phenotypic classes in gpr56 stl13/stl13 mutants such that the majority (76%) of gpr56 stl13/stl13 larvae expressed WT levels of mbp ( Fig. 7i , N=13/17). Importantly, all embryos analysed for these studies were morphologically normal, and thus changes in mbp expression could not be attributed to changes in overall heath in treated animals compared with controls ( Fig. 7g,h,k and l ). Taken together, these experiments demonstrate that Gpr56 interacts with Gα 12/13 and signals through RhoA to promote oligodendrocyte development and subsequent myelination. The timing of the transition from OPC proliferation to terminal differentiation is tightly regulated [40] , [41] , [42] . In the CNS, interactions between receptors on the OPC cell surface and axon-bound or axon-secreted molecules ensure that sufficient numbers of OPCs are generated to accommodate the numbers of axons that need to be myelinated. Availability of the axon-derived mitogen PDGF-A, which interacts with PDGFRα on the OPC plasma membrane, is a major determinant of the extent of OPC proliferation. Moreover, numerous mechanisms converge to ensure the timing and execution of terminal differentiation, including downregulation of Pdgfr α by Nkx2.2 in OPCs, cell-cycle exit and vast morphological changes [37] , [42] , [43] , [44] , [45] . Failed differentiation of resident OPC pools in response to demyelination is a major contributor to the degenerative nature of demyelinating diseases such as multiple sclerosis [46] ; thus, identification of signalling molecules that regulate OPC behaviour and differentiation could provide new avenues for therapeutics. In this study, using zebrafish and mouse models, we identified Gpr56 as a new regulator of OPC proliferation and oligodendrocyte myelination. Like PDGFRα, Gpr56 expression is restricted to early stages of oligodendrocyte development and is downregulated before terminal differentiation [18] , [42] , suggesting that Gpr56 may negatively regulate terminal differentiation and/or positively regulate OPC behaviour/proliferation. Gpr17, another GPCR that is essential for oligodendrocyte development, is also expressed in OPCs and is downregulated in mature oligodendrocytes, and Gpr17 has been shown to directly inhibit terminal differentiation. In the absence of Gpr17 , OPCs prematurely differentiate and form myelin, though myelination eventually proceeds to WT levels in Gpr17−/− mice [47] . We found that gpr56 stl13/stl13 mutant OPCs likewise formed associations with axons and myelinated prematurely, indicative of precocious differentiation due to relieved inhibition on terminal differentiation. We found that OPCs are specified normally in gpr56 stl13/stl13 mutants but are less proliferative, resulting in reduced numbers of myelinating oligodendrocytes and consequently hypomyelination. In addition, transient OE of gpr56 in WT embryos caused increased numbers of pro-OLs and increased mbp expression in gpr56 OE embryos at 2.5 dpf. However, the apparent increase in mbp expression is likely the result of greater numbers of pro-OLs, as myelination was inhibited in the OE embryos at 5 dpf as assessed by TEM. We also observed many immature oligodendrocyte cell bodies with no axonal contacts in the centre of the spinal cord of the OE embryos at this time point. These findings indicate that the prolonged OE of gpr56 inhibits OPC differentiation and myelination. Together, these findings support the hypothesis that Gpr56 is both a positive regulator of OPC proliferation and an inhibitor of oligodendrocyte terminal differentiation. Though we observed striking defects in oligodendrocyte development and myelination when Gpr56 function is perturbed, we did not observe any defects in the development of neurons, radial glia or in microglia number in gpr56 stl13/stl13 mutants at any time point analysed. These data suggest that the observed defects in oligodendrocyte development are a cell-autonomous effect, although conditional mouse mutant studies could be leveraged to definitively address the question of cellular autonomy. Together, these data demonstrate that Gpr56 is a positive regulator of OPC proliferation and a negative regulator of OPC differentiation. Previous in vitro studies place Gα 12/13 and RhoA signalling downstream of Gpr56 (refs 35 , 36 ). RhoA is the major downstream effector of Gα 12/13 and its expression is likewise restricted to early stages of oligodendrocyte development [37] , [39] . Inactivation of RhoA via Fyn is required for OPC morphological differentiation into pro-OLs, and sustained OE of RhoA inhibits process extension and differentiation of oligodendrocytes [37] . Reduction of Gα 12/13 function in gpr56 stl13/stl13 zebrafish mutants and heterozygotes causes enhanced loss of CNS mbp expression. In addition, transient OE of constitutively active RhoA before terminal differentiation suppressed gpr56 stl13/stl13 defects. In sum, these data support a model in which Gpr56 function in OPCs is mediated via interactions with Gα 12/13 and RhoA signalling. RhoA has not been shown to directly promote OPC proliferation, though our findings do not preclude this possibility. We therefore propose a model in which Gpr56 interacts with Gα 12/13 and activates RhoA to prevent OPC differentiation, which facilitates continued OPC proliferation promoted by axon–glia interactions such as those mediated by PDGFRα and PDGF-A [42] , [43] , [44] . When Gpr56 function is perturbed, RhoA activation is therefore reduced, relieving RhoA inhibition of terminal differentiation and causing premature OPC differentiation that manifests in a reduced proliferation phenotype ( Fig. 8 ). In this model, the OPCs that prematurely undergo terminal differentiation should myelinate normally. Accordingly, we detected an increase in axons associated with pro-OLs at 30 hpf and increased myelination at 3 dpf, consistent with precocious differentiation. Furthermore, we observed no myelin abnormalities or reduced myelin thickness in those axons that are myelinated in gpr56 stl13/stl13 mutants. In sum, these data support the model that Gpr56 positively regulates OPC proliferation via RhoA activation and inhibition of terminal differentiation. 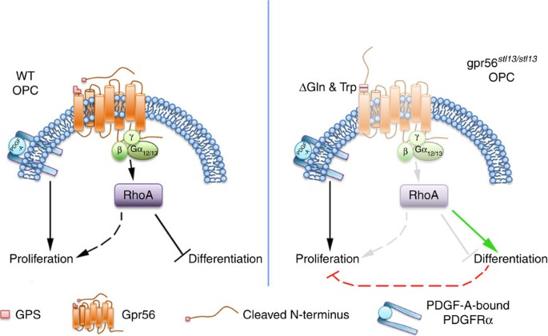Figure 8: Gpr56 promotes OPC proliferation through inhibiting differentiation. Model of Gpr56 function in OPCs. In WT OPCs, Gpr56 couples to Gα12/13and activates RhoA, which prevents terminal differentiation and indirectly promotes OPC proliferation (dashed arrow) by maintaining the OPC in an immature, proliferative state. OPC proliferation is directly regulated via interactions between neuron-secreted PDGF-A and OPC-bound PDGFRα. In Gpr56 (stl13/stl13) mutant OPCs, impaired autoproteolytic cleavage reduces Gpr56 signalling capacity, leading to loss of RhoA activation. Reduced RhoA signalling alleviates RhoA inhibition on terminal differentiation (green arrow), which indirectly causes a decrease in OPC proliferation (red dashed lines) as OPCs differentiate at the expense of proliferation. Figure 8: Gpr56 promotes OPC proliferation through inhibiting differentiation. Model of Gpr56 function in OPCs. In WT OPCs, Gpr56 couples to Gα 12/13 and activates RhoA, which prevents terminal differentiation and indirectly promotes OPC proliferation (dashed arrow) by maintaining the OPC in an immature, proliferative state. OPC proliferation is directly regulated via interactions between neuron-secreted PDGF-A and OPC-bound PDGFRα. In Gpr56 ( stl13/stl13 ) mutant OPCs, impaired autoproteolytic cleavage reduces Gpr56 signalling capacity, leading to loss of RhoA activation. Reduced RhoA signalling alleviates RhoA inhibition on terminal differentiation (green arrow), which indirectly causes a decrease in OPC proliferation (red dashed lines) as OPCs differentiate at the expense of proliferation. Full size image At present, multiple ligands of Gpr56 have been identified in other cell types. In cancer studies, Gpr56 has been shown to inhibit melanoma cell growth via interactions with tissue transglutaminase (TG2) [48] . In the developing brain, collagen type III, alpha-1 secreted by meningeal fibroblasts interacts with neuron-bound Gpr56 to facilitate proper neuronal migration [36] . Impaired differentiation of OPC progenitors is a major cause of failed remyelination in the CNS of patients suffering from demyelinating diseases such as multiple sclerosis [46] . Therefore, a better understanding of Gpr56 activation and signalling is crucial as targeted inhibition of this receptor could be used to promote OPC differentiation and remyelination after injury and disease-induced demyelination. Further studies are required to identify the endogenous ligand(s) and small molecules that modulate Gpr56 signalling in OPCs. Zebrafish stocks and rearing conditions Zebrafish ( Danio rerio ) were maintained in the Washington University Zebrafish Consortium facility ( http://zebrafish.wustl.edu/husbandry.htm ). All experiments were performed in compliance with Washington University’s institutional animal protocols. Embryos were collected from pair-wise or harem matings and reared at 28.5 °C in egg water (5 mM NaCl, 0.17 mM KCl, 0.33 mM CaCl 2 , 0.33 mM MgSO 4 ). Embryos were staged in hours post-fertilization (hpf) or days post-fertilization (dpf) using morpholical markers [49] . To prevent pigmentation in embryos >1 dpf, egg water was supplemented with phenylthiourea to 0.003%. The following lines of zebrafish were used for these studies: both alleles of gpr56 ( stl13, stl14 ) were generated in a WT (AB*) background. For marker analysis, we used the following transgenic lines: tg ( gfap:GFP ) [50] , tg(sox10(−7.2):mRFP) [24] , tg(olig2:dsred) [51] , tg(HuC:kaede) [52] and tg(sox10(−7.2):memgfp ) that were a generous gift from Mark Voigt (St. Louis University). Genotyping To genotype individual larvae for phenotypic analyses, we used the following primers to amplify a 182 bp fragment of gpr56 from genomic DNA: 5′- CATGGGATACAAAACAAGGT -3′ and 5′- AGTGGCATTCTGTCTGTTCT -3′. For stl14 , PCR products were run out on a 3% agarose gel and the smaller fragment (158 bp) is the mutant allele. For stl13 , we performed restriction digest analysis using Hpy166II, which cleaves WT into a 61 bp and a 121 bp fragment, but is unable to cut mutant (176 bp). TALEN generation and microinjection: TALEN constructs were assembled by the Hope Center for Neurological Disorders at Washington University using the Golden Gate TALEN assembly protocol [53] . The repeat variable diresidue sequences for the left and right TALENs were as follows: Left : NN NG NG NG HD NG HD HD HD NG NI NN NI HD NI NI NG and Right : NI NI HD NG NN NG NI NG HD NN HD NI NN HD HD NI NG HD NI NG. Synthetic TALEN mRNA was then transcribed using the mMESSAGE mMACHINE SP6 ULTRA kit (Ambion), and RNA from each arm was combined and injected into single-cell stage WT embryos (AB) at 100 pg quantities. To recover germ-line transmitted mutations, injected founders (F0s) were raised to adulthood, outcrossed to WT AB partners, and genomic DNA was extracted from individual F1 embryos for PCR amplification and restriction digest analysis of the targeted region. Genomic DNA from F1 embryos that showed disruption of the target site was then cloned using the TOPO TA Cloning kit (Invitrogen) and sequenced using Sanger sequencing. Mice All mouse ( Mus musculus ) experiments were performed in compliance with Washington University’s institutional animal protocols. The Gpr56 -knockout mice were obtained from the Mutant Mouse Regional Resource Centers (MMRRC), were maintained on a C57BL/6 background and genotyped as described previously [29] . P3 animals of presumed mixed gender were used for all neurosphere experiments, although pups were not genotyped for gender. PCR with reverse transcription Standard PCR with reverse transcription (RT–PCR) was performed on cDNAs derived from embryos at the two-cell stage (Maternal), 8 hpf, 24 hpf, 48 hpf, 72 hpf and 5 dpf. Analysis was performed three separate times with similar results. For all stages, cDNA was reverse-transcribed from RNA extracted from pools of 30 embryos with the SuperScript First-Strand Synthesis system for RT–PCR (Invitrogen) using Superscript II reverse transcriptase (RT) and oligo(dT) primers, and genomic DNA was controlled for by omitting RT from reactions using the same RNA. To amplify gpr56 , we used primers that amplify a 602-bp fragment from exons 3 to 7: 5′- TCATCCAGAAGAGCTGATTT -3′ and 5′- GAAATTTCAGCCAATGAGAG -3′. gapdh was amplified as a control to produce a 117-bp product: 5′- TGACCCATTCATTGACCTTG -3′ and 5′- GCATGACCATCAATGACCAG -3′. Cloning Full-length gpr56 cDNA was amplified from cDNA derived from 5 dpf embryos and cloned into pCS2+ using the following primer set: 5′- GATCTA CTCGAG TTGGTAGAAAGTGGACTTCG -3′ (XhoI site underlined) and 5′- AGGATA TCTAGA TTCCCTCACAACTTCACACT -3′ (XbaI site underlined). Both vector and insert were digested with XhoI and XbaI and ligated together using standard T4 ligase (NEB), and the final vector (pCS2+_ zf_ gpr56 ) was sequenced for verification. In situ hybridization Whole-mount in situ hybridizations were performed using standard protocols [54] . In brief, embryos were fixed at the desired age with 4% paraformaldehyde for 2 h at room temperature or 4 °C overnight, and then dehydrated in 100% Methanol overnight. Following dehydration, embryos were washed in 0.2% PBS-Tween (PBSTw), permeabilized in proteinase K (20 mg μl −1 diluted 1:1,000 in 0.2% PBSTw), and incubated with the appropriate Digoxygenin-labelled riboprobe overnight at 65 °C in hybridization buffer (50% formamide). Following probe treatment, embryos were washed to remove formamide, blocked in 2% blocking medium supplemented with 10% normal sheep serum and 0.2% Triton, and incubated in the primary antibody (Anti-Dig, Fab fragments (1:2,000), Roche) overnight in a block. Following primary antibody treatment, embryos were washed in Maleic Acid Buffer with 0.2% Triton and developed by alkaline phosphatase treatment. When complete, embryos were post-fixed in 4% paraformaldehyde and stored long-term in 70% glycerol. To synthesize gpr56 riboprobes, a 509-bp region spanning exons 11–13 was PCR amplified from a partially sequenced cDNA clone (Clone ID 7070653, Open Biosystems) using the following primer pair: 5′- ATTTCTGCTGTGCTTGTTCT -3′ and 5- CATGTGGTTCCATACAGACA -3′. The PCR product was cloned into pCR II using the pCR II- TOPO TA Cloning kit (Invitrogen) and sequenced. This construct was linearized by NotI and transcribed with SP6 for sense and linearized with BamHI and transcribed with T7 for antisense. All other riboprobes: mbp [55] , nkx2.2a [56] , apoeb [57] , shh [58] , ptc1 (ref. 59 ) and ptc2 (ref. 60 ) were described previously. Embryos stained with nkx2.2a were mounted in glycerol and nkx2.2a positive cells were counted manually in all focal planes of the spinal cord from segments 5–7 or 15–30. apoeb positive microglia were counted as previously described [57] . All quantifications were performed blinded, and genotypes were obtained following quantification. Transmission electron microscopy For zebrafish larvae and 21 dpf juveniles, TEM was performed using a PELCO BioWave Pro with SteadyTemp Digital Plus water-recirculating system to ensure sufficient infiltration of the embryos [61] . Embryos were microwaved for all steps before EPON treatment. In brief, embryos were fixed in Karnovsky’s fix (4% paraformaldehyde, 2% glutaraldehyde, 0.1 M sodium cacodylate) and left overnight at 4 °C. After fixation, embryos were post-fixed in 2% osmium tetroxide in 0.1 M sodium cacodylate and 0.1 M imidazole, washed and treated with saturated uranyl acetate. Embryos were then dehydrated using increasing concentrations of ethanol followed by 100% acetone, and then infiltrated overnight in an acetone-EPON mixture. Embryos were then transferred to 100% EPON and embedded in moulds for baking overnight at 65 °C. We always examined fish of a given stage at approximately the same body segment level to control for variability along the anterior/posterior axis. For preparation of spinal cords from 6–month- old adults, we anaesthetized animals in an ice-water bath and then severed the hindbrain before dissecting a portion of the anterior spinal cord, and fixation of adult-tissue occurred as described previously [10] . In brief, adult tissues were fixed in Karnovsky’s fix overnight, post-fixed in 2% osmium tetroxide in 0.1 M sodium cacodylate, washed and dehydrated in increasing concentrations of ethanol followed by 100% propylene oxide. The tissues were then submerged in a 2:1 mixture of propolyene oxide:EPON for 1 h, followed by a 1:1 mixture overnight. The following day, the tissues were transferred to 100% EPON before embedding and baking at 65 °C. Thin sections (70 nm) were mounted on mesh (5 dpf and 6 month samples) or slot (21 dpf samples) grids and stained with 8% uranyl acetate and Sato’s lead stain. Sections were then viewed on a Jeol (JEM-1400) electron microscope and images were collected with an AMT V601 digital camera. All images were processed and analysed using Image J software. At 3 and 5 dpf, quantifications were performed on a stereotyped, 14 μm 2 region of the dorsal or ventral spinal cord containing ~400 and 250 axons, respectively (see Fig. 3b ). At 21 dpf, quantifications were performed on three, 20 μm 2 sections of the ventral spinal cord and two, 20 μm 2 sections of the dorsal spinal cord containing of a minimum of 100 and 300 axons, respectively. Quantifications were performed on stereotyped positions of the spinal cord (see Fig. 3b ). At 6 months, quantifications were performed on a stereotyped 17 μm 2 region of the dorsal and ventral spinal cord ( Supplementary Fig. 7a ). G-ratios were calculated using Adobe Photoshop and Image J software for ~50 axons per animal by taking the ratio of the axon diameter to the diameter of the whole myelinated fibre. At 3 dpf, N =3 for WT and gpr56 stl13/+ , N =4 for gpr56 stl13/stl13 . For quantification of gpr56 mutants and controls at 5 dpf, N =6 for WT controls, N =5 for gpr56 stl13/stl13 mutants and N =4 for gpr56 stl14/stl14 mutants. At 21 dpf, N =2 for WT controls and N =4 for gpr56 stl13/stl13 mutants. At 6 months, N =3 for WT controls and N =4 for gpr56 stl13/stl13 mutants. For quantification of gpr56 -injected versus control-injected embryos at 2.5 and 5 dpf, we manually counted the number of wraps around Mauthner axons imaged at × 10,000. At 2.5 dpf, we quantified all neuronal/oligodendrocyte-lineage cell bodies in the dorsal half of the spinal cord (located above half the height of the whole spinal cord at × 1,200). N =4 for each treatment. At 5 dpf ( N =4 for control-injected embryos, N =5 for gpr56 -injected embryos), we quantified oligodendrocyte-lineage cell bodies within a stereotyped 30 μm 2 region in the centre of the spinal cord. Additional calculations were performed as described above. All quantifications were performed blinded to genotype and treatment. Culture and generation of neurospheres For generation of neurospheres for IHC analysis, spinal cords and subventricular zones (SVZ) were dissected from postnatal (P) day 3 mice ( Gpr56+/+ : N =3; Gpr56+/− : N =4; Gpr56−/− : N =5) to generate NPCs as previously reported [62] . In brief, spinal cords and SVZ were removed from P3 mice and processed to obtain single-cell suspension of neural progenitors (neurospheres). Dissected spinal cords and SVZ were digested with trypsin digest buffer containing 0.2% BSA (Sigma), 0.5 mg ml −1 DNase I (Sigma) and 10% trypsin-EDTA stock (BioWhittaker) in HBSS at 37 °C for 15 min in a volume of 0.7 ml l −1 . Equal volumes of 10% FBS medium containing 10% FBS (Life Technologies) and low glucose DMEM (Sigma) were added, and spinal cords and SVZ were triturated with fire-polished Pasteur pipettes. Pelleted cells were washed with dissociation medium containing 15 mM HEPES (Sigma), 0.5% glucose in HBSS. Cells were finally resuspended in NSC medium containing a 5:3 mixture of DMEM low glucose:Neurobasal medium (Life Technologies), 0.5 mM 2-mercaptoethanol, 2 mM L-glutamine, 5 IU of penicillin and 5 μg ml −1 streptomycin (BioWhittaker) supplemented with 1% N2 supplement (Life Technologies), 2% B27 supplement (Life Technologies), 20 ng ml −1 epidermal growth factor (EGF) (Sigma) and 20 ng ml −1 basic fibroblast growth factor (FGF) (R & D Systems). Cells were allowed to grow in culture for 6 days. For generation of neurospheres for western blotting analysis, SVZ were dissected from P3 mice ( Gpr56+/+ : N =4; Gpr56+/− : N =4; Gpr56−/− : N =3) and cultured as described above. Neurosphere immunocytochemistry Immunocytochemistry was performed on trypsinized NPCs grown in 50 μg ml −1 poly- D -lysine-coated and 10 μg ml −1 fibronectin-coated 24-well plates containing defined medium [(5:3 mixture of DMEM low glucose (Life Technologies): neurobasal medium (Life Technologies), 0.5 mM 2-mercaptoethanol, 2 mM L -glutamine, 5 IU of penicillin and 5 μg ml −1 streptomycin (Life technologies) supplemented with 1% N2 supplement (Life Technologies) and 2% B27 supplement (Life Technologies) without growth factors. After 5 days in culture, cells were fixed and stained with primary antibodies (Nestin: ab6142 (Abcam), GFAP: G9269 (Sigma-Aldrich), Tuj1: MMS-435P (Covance) and O4: MAB345 (Millipore)) at 4 °C overnight. For fluorescence detection, Alexa Fluor-tagged secondary antibodies (Molecular Probes) were used and cells were counterstained with DAPI. Images were acquired using Metamorph software on a Nikon Eclipse TE300 microscope equipped with an optical camera (Optronics). Investigators were blinded to mouse genotypes and percentages of positive cells were calculated using the total number of cells in each image (DAPI nuclear stain). Data were analysed with Prism 5 software (GraphPad Software) using a two-way ANOVA test as all data met the common assumptions (normally distributed, equal variances, independent samples) required for this test. Neurosphere western blotting Western blots were performed as previously described [62] . Images of full western blots can be seen in Supplementary Figs 8 and 12 . In brief, neurospheres were lysed in MAPK lysis buffer (20 mM Tris [pH 7.0], 10 mM EGTA, 400 mM B -glycerophosphate, 1% NP-40, 2.5 mM MgCl 2 and 2 mM sodium orthovanadate with protease inhibitors (leupeptin, aprotinin and phenylmethylsulfonyl fluoride). Proteins were separated by SDS–polyacrylamide gel electrophoresis (SDS–PAGE) and transferred to polyvinylidene difluoride membranes (Millipore) before detection with phospho-specific antibodies. Antibodies that detect the total expression of the corresponding signalling intermediate (Gpr56-H11 (1:1,000) [63] ; RhoA (1:1,000): #2117, Cell Signaling) as well as α-tubulin ((1:30,000), T745, Sigma) were used as controls for equal protein loading and quantitation. Active RhoA (RhoA-GTP) was determined by PAK1-PBD affinity chromatography ((1:200), M17-294, Millipore) according to the manufacturer’s recommendations. Appropriate HRP-conjugated secondary antibodies (anti-rabbit (1:5,000): 7074 and anti-mouse (1:5,000): 7076, Cell Signaling) were used for detection by enhanced chemiluminescence (New England Biolabs). Time-lapse imaging Embryos were mounted in 1% low melting agarose with tricaine to prevent movement and 0.003% phenylthiourea to prevent pigmentation. Embryos were oriented laterally and all images were taken of spinal cord regions spanning segments 5–7 using a × 40 dry objective. Time-lapse images were taken from gpr56 stl13/stl13 mutants ( N =7) and gpr56 stl13/+ controls ( N =6) expressing tg(sox10:mRFP ) [24] from 30 to 46 hpf using a Quorum spinning disc confocal microscope on a heated stage, recorded using Metamorph software, and analysed using Image J. All analyses were performed blinded to genotype. Zebrafish immunohistochemistry and fluorescence imaging For imaging of transgenes in fixed embryos, embryos were fixed in fresh, 4% paraformaldehyde supplemented with 0.1 M pipes, 1.0 mM MgSO 4 , and 2 mM EGTA in 1 × PBS to preserve fluorescence [64] . For phospho-H3 antibody stains (06570MI, Millipore), embryos were fixed in 4% paraformaldehyde in 1 × PBS overnight (4 °C), washed in 0.3% PBS/Triton and then blocked for 2 h in 0.3% PBS/Triton plus 10% normal goat serum and 4% BSA. Embryos were then incubated overnight at 4 °C in primary diluted 1:3,000 in blocking solution. For secondary staining, embryos were incubated in Alexa Flour goat anti-rabbit 488 IgG (Life Technologies) diluted 1:2,000 in 0.3% PBS/Triton plus 2% normal goat serum for 3 h at room temperature. Finally, embryos were washed and mounted in vectashield (Vector Labs) for imaging. All quantifications were performed blinded, and genotypes were obtained following quantification. Morpholino and synthetic mRNA injections The morpholinos targeting gna12 , gna13a and gna13b are previously published [38] and were a kind gift from Fang Lin (University of Iowa). Morpholinos were combined and diluted in sterile water supplemented 1:10 with phenol-red dye, and then injected at a final concentration of 1 ng each in a total volume of 1 nl. To control for adverse side-effects from the injection process, we also injected control siblings with an equal volume of phenol-red diluted 1:10 in water. Contstitutively active Rho ( rhoV14 ) was kindly provided by Lila Solnica-Krezel and was transcribed and injected as described previously [38] . The full-length mouse Gpr56 cDNA clone was obtained from Open Biosystems (Clone ID: 3709247), linearized with NotI, transcribed using the mMESSAGE mMACHINE SP6 ULTRA kit (Ambion) and injected at a final concentration of 200 pg in 2 nl. For transcription of pCS2+_ zf _gpr56 , the plasmid was linearized with NotI and also transcribed using the mMESSAGE mMACHINE SP6 ULTRA kit (Ambion) before injection of a total concentration of 50 pg in 3 nl. Statistical analyses All data are presented as the mean+or±s.d. To represent significance: *, P <0.05; **, P <0.01; ***, P <0.001, a minimum of two technical replicates were performed for each described experiment unless noted otherwise. Although we did not perform statistical tests to predetermine sample size, our sample sizes are similar to previously published studies. For cell-count, molecular marker and time-lapse imaging analyses in zebrafish, a minimum of six animals per genotype were used for each described marker, which is in line with previously published works [10] , [55] , [57] . Similarly, for TEM analyses, a minimum of two WT and four mutant animals were analysed at each developmental stage as previously described [10] , [34] . For neurosphere studies, we used at least three animals per genotype, and for IHC experiments cell counts were taken from three nonadjacent sections of each well in triplicate [62] . Finally, for injection studies, a minimum of 10 animals were analysed per genotype and treatment group, similar to previously published studies [10] , [55] . Unless otherwise noted, statistical analyses were performed using an unpaired Student’s t -test with two tails, unequal variance. With few exceptions, all data sets analysed by a Student’s t -test met the appropriate assumptions, including normality. All data sets with a skewness and kurtosis with an absolute value of ≤1 were considered approximately normal. The data sets that did not follow a normal distribution were represented by the following graphs: Figs 3o , 7j , and Supplementary Fig. 3i . These data sets showed low variability, causing a kurtosis value of >1. Because the mean and s.d. values were nearly identical between both control and experimental groups for these experiments, and we found no significant difference between these groups using the student’s t -test, we did not feel that the test was inappropriate for these analyses. How to cite this article : Ackerman, S. D. et al . The adhesion GPCR Gpr56 regulates oligodendrocyte development via interactions with Gα 12/13 and RhoA. Nat. Commun. 6:6122 doi: 10.1038/ncomms7122 (2015).